Experimental measurement-device-independent verification of quantum steering Bell non-locality between distant quantum systems—that is, joint correlations which violate a Bell inequality—can be verified without trusting the measurement devices used, nor those performing the measurements. This leads to unconditionally secure protocols for quantum information tasks such as cryptographic key distribution. However, complete verification of Bell non-locality requires high detection efficiencies, and is not robust to typical transmission losses over long distances. In contrast, quantum or Einstein–Podolsky–Rosen steering, a weaker form of quantum correlation, can be verified for arbitrarily low detection efficiencies and high losses. The cost is that current steering-verification protocols require complete trust in one of the measurement devices and its operator, allowing only one-sided secure key distribution. Here we present measurement-device-independent steering protocols that remove this need for trust, even when Bell non-locality is not present. We experimentally demonstrate this principle for singlet states and states that do not violate a Bell inequality. Entanglement provides a fundamental resource for a range of quantum technologies, from quantum information processing to enhanced precision measurement [1] , [2] , [3] , [4] . In particular, the strong correlations inherent in shared entanglement—for example, between two parties—allows secure messaging and quantum information transfer, potentially over long distances [1] , [5] . At the same time, the strong restrictions of quantum measurement theory prevents the extraction of useful information when an adversary has access to only one of the entangled systems [6] , [7] , [8] . Furthermore, any adversary measuring one or more of the entangled systems reveals their presence to the communicating parties. When correlations due to quantum entanglement are sufficiently strong, they allow the unconditionally secure sharing of a cryptographic key between two distant locations, without requiring any trust in the devices used or in the observers reporting the results [9] . They also allow generation of unconditionally genuine randomness, again with no trust in the devices used or their operators [10] , [11] . The corresponding verification protocols are thus device-independent, and can be put in the form of a ‘Bell-non-local game’, played between a referee and two untrusted parties, which can be won by the latter only if they genuinely share a Bell-non-local quantum state ( Fig. 1a ) [12] , that is, an entangled state that violates a Bell inequality. 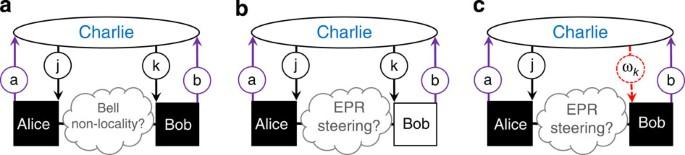Figure 1: Quantum correlation games. (a) In ‘non-local games’ a referee (Charlie) can verify that Alice and Bob share a Bell-non-local resource, by sending classical input signalsjandk, receiving output signalsaandband checking whether the corresponding correlations violate a Bell inequality. No trust in Alice and Bob or their devices is necessary, as indicated by the black boxes. (b) The referee may similarly use an ‘EPR steering game’ to verify the presence of an EPR steering resource, by checking whether the correlations violate a suitable EPR steering inequality. However, all known EPR steering games require the referee to fully trust one of the observers and their devices, as indicated by the transparent box. (c) Using the measurement-device-independent protocols of this paper, the referee can now unconditionally verify EPR steering, by using ‘quantum-refereed steering games’ that replace the need for trust with quantum input signalsωk. Figure 1: Quantum correlation games. ( a ) In ‘non-local games’ a referee (Charlie) can verify that Alice and Bob share a Bell-non-local resource, by sending classical input signals j and k , receiving output signals a and b and checking whether the corresponding correlations violate a Bell inequality. No trust in Alice and Bob or their devices is necessary, as indicated by the black boxes. ( b ) The referee may similarly use an ‘EPR steering game’ to verify the presence of an EPR steering resource, by checking whether the correlations violate a suitable EPR steering inequality. However, all known EPR steering games require the referee to fully trust one of the observers and their devices, as indicated by the transparent box. ( c ) Using the measurement-device-independent protocols of this paper, the referee can now unconditionally verify EPR steering, by using ‘quantum-refereed steering games’ that replace the need for trust with quantum input signals ω k . Full size image There are, however, practical difficulties in entanglement verification via Bell-non-local games. Even if the entanglement is strong enough (compared with noise) to otherwise violate a Bell inequality, there may be too many null measurement results for unconditional verification—arising, for example, from detector inefficiencies or the typical transmission losses involved in implementations over long distances. Too many null results will make it impossible even for ‘honest’ devices to win a Bell-non-local game. This is the well-known ‘detection loophole’ [13] . A promising alternative is based on a different test of non-locality, called Einstein–Podolsky–Rosen (EPR) steering (or quantum steering). First identified by Erwin Schrödinger [14] , and present in the EPR paradox [15] , this corresponds to being able to use entanglement to steer the state of a distant quantum system by local measurements, and is strictly weaker than Bell non-locality [16] , [17] . Further, the detection loophole can be circumvented in the verification of steering, if the device and operator for one of the two entangled systems is completely trusted by the referee [18] , [19] , [20] ( Fig. 1b ). This leads to the real possibility of one-sided device-independent secure key distribution that is robust to both detector inefficiency and transmission loss [21] . Unfortunately, however, an unconditionally secure protocol cannot rely on trust at all, even in one side. Very recently, work on entanglement verification by Buscemi [22] has been generalized to show that EPR steering can in fact be verified in the absence of trust in either side, via quantum-refereed steering (QRS) games [23] . In comparison with Bell-non-local games, the referee still sends classical signals to one party, but sends quantum signals to the other party ( Fig. 1c ). The quantum signals must be chosen such that they cannot be unambiguously distinguished, to prevent the possibility of cheating. Until now, only an existence proof for such games was known, with no explicit means of construction [23] . For the case of entanglement witnesses, a recent measurement-device-independent protocol and demonstration has addressed a similar question [24] , [25] , although EPR steering, Bell non-locality and calibration of the quantum signals (see below) were not considered. In this paper we give the first explicit construction of a QRS game, for the trust-free verification of steering entanglement. We also demonstrate a proof-of-principle implementation, for optical polarization qubits, in a scenario where no Bell non-locality—as tested by the Clauser–Horne–Shimony–Holt (CHSH) inequality [26] —is present. The results open the way to measurement-device-independent key distribution protocols that do not require Bell non-locality, and which can circumvent the detection loophole. Quantum-refereed steering game Consider the following scenario ( Fig. 1c ). On each run the referee, whom we shall call Charlie, chooses at random a pair of numbers labelled by k ≡( j , s ), with j ε{1, 2, 3} and s =±1. Charlie sends Alice the value of j as a classical signal, and sends Bob a qubit in the s -eigenstate of the Pauli spin observable , that is, the state . The referee requires Alice and Bob to send back classical binary signals, a =±1 and b =0 or 1, respectively. The referee uses their reported results over many runs to calculate the payoff function where ‹·› j , s denotes the average over those runs with k =( j , s ). Here r ≥1 is a parameter that indicates how well the referee can prepare the desired qubit states , with r =1 for perfect preparation (see Methods section). Alice and Bob win the game if and only if P ( r )>0. In this QRS game Alice and Bob are allowed to plan a joint strategy beforehand, but are not allowed to communicate during the game. The latter could be enforced via space-like separated measurement regions. The game is measurement-device-independent, because Charlie makes no assumptions about how Alice and Bob generate their values of a and b —they and their devices are untrusted. Remarkably, Alice and Bob cannot cheat—they are only able to win the game if Alice is genuinely able to steer Bob’s state (see Methods section). For example, suppose that Alice and Bob share a two-qubit Werner state, , where 0≤ W ≤1 and |Ψ − › AB denotes the singlet state [27] , and adopt the following strategy: on receipt of signal j Alice measures , while Bob measures the projection operator |Ψ − › BC ‹Ψ − | onto the singlet state in the two-qubit Hilbert space spanned by his system and . It is straightforward to calculate that the corresponding theoretical value of the payoff function in equation (1) is Hence Alice and Bob can, in principle, win the game whenever . This condition is in fact necessary for them to be able to win the game with a shared Werner state (see Methods section), and therefore the above strategy is optimal. A QRS game can be constructed for every quantum state that is EPR steerable (see Methods). Quantum signals must be sent to Bob if it is to be verified that Alice can steer Bob’s state, and to Alice if the converse is to be verified. Note this directionality of EPR steering is non-trivial: for some quantum states only one-way EPR steering is possible [28] , [29] , [30] . Measurement-device-independent verification of EPR steering We experimentally verified device-independent EPR steering using our quantum-refereed game. Alice and Bob’s shared state, and the states sent by Charlie to Bob, were encoded in photon polarization qubit states. The payoff function P ( r ) was calculated via single-qubit measurements and a partial Bell-state measurement (BSM), all using linear optics and photon counting ( Fig. 2 ) [31] . 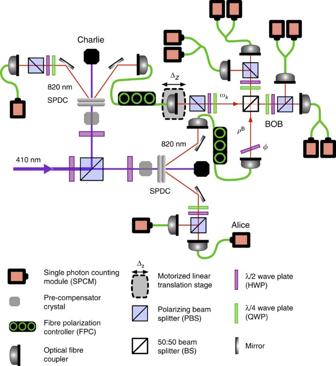Figure 2: Illustration of experimental apparatus. A pair of separate spontaneous parametric down-conversion (SPDC) sources create Alice’s, Bob’s and Charlie’s photons. One photon from Charlie’s source acts as a heralding signal, with the remaining photon prepared in the quantum stateωkand sent via optical fibre to the input of Bob’s partial BSM device, accompanied by a corresponding classical signaljε{1, 2, 3} sent to Alice. Using a 50:50 beam splitter, Bob combines Charlie’s photon (prepared in stateωk) with his own photonρB(comprising half of the entangled stateρABshared with Alice), and projects onto the singlet subspace |Ψ−BC›‹Ψ−BC|. Alice receives Charlie’s announcementjaccompanied by the other half of the shared entangled stateρAB, and measuresσj. To execute the entanglement verification, Charlie receives Alice’s and Bob’s output signalsaε{±1} andbε{0, 1}, and computes a payoff functionP, whereP>0 witnesses quantum steering in a device-independent setting. Figure 2: Illustration of experimental apparatus. A pair of separate spontaneous parametric down-conversion (SPDC) sources create Alice’s, Bob’s and Charlie’s photons. One photon from Charlie’s source acts as a heralding signal, with the remaining photon prepared in the quantum state ω k and sent via optical fibre to the input of Bob’s partial BSM device, accompanied by a corresponding classical signal j ε{1, 2, 3} sent to Alice. Using a 50:50 beam splitter, Bob combines Charlie’s photon (prepared in state ω k ) with his own photon ρ B (comprising half of the entangled state ρ AB shared with Alice), and projects onto the singlet subspace |Ψ − BC ›‹Ψ − BC |. Alice receives Charlie’s announcement j accompanied by the other half of the shared entangled state ρ AB , and measures σ j . To execute the entanglement verification, Charlie receives Alice’s and Bob’s output signals a ε{±1} and b ε{0, 1}, and computes a payoff function P , where P >0 witnesses quantum steering in a device-independent setting. Full size image The QRS game requires two components: the entanglement shared between Alice and Bob and the qubit encoding the state ω k from Charlie. These were generated using a degenerate 820 nm polarization entanglement source, and a heralded single-photon source at 820 nm, respectively. To play the game, different measurement apparatus is required for Alice and Bob: Alice only makes single-qubit measurements, while Bob implements a two-qubit measurement between his half of the entangled pair, and the incoming qubit from Charlie. This two-qubit measurement was implemented using a partial BSM device. Thus, Bob implemented projections onto the singlet subspace |Ψ − › BC ‹Ψ − | (corresponding to the outcome b =1) and the triplet subspace (−|Ψ − › BC ‹Ψ − |) (corresponding to b =0), of the two-qubit Hilbert space spanned by his and Charlie’s systems (see Methods). However, the inner workings of Alice and Bob’s apparatus need not be known, because the protocol is measurement-device-independent. In particular, a key innovation of our protocol is that the payoff function P ( r ) in equation (1) cannot present ‘false positives’ of EPR steering. Alice and Bob do not have to be trusted and can try to cheat by any means, provided that they cannot communicate during the demonstration. This result requires r ≥ r * in the payoff function P ( r ) to assure measurement-device independence, where r * characterizes the quality of Charlie’s preparation of the states he sends to Bob ( r *≥1, r *=1 perfect; see Methods). In this work we choose r = r *. To implement our protocol, Charlie sent Bob a qubit ω k (derived from the heralded single-photon source) encoded in the , , or basis, and announced to Alice a corresponding value of j =1, 2 or 3. Alice implemented a measurement on her half of the entangled state (projective, in the , or basis depending on Charlie’s announcement) and Bob implemented his partial BSM. Charlie received classical outputs from Alice ( a =±1) and Bob ( b =0 or 1) over many runs. Using this information Charlie calculated the payoff function P ( r ) in equation (1), and tested for positivity to verify EPR steerability. We tested for device-independent steering both for highly entangled states and also in the regime where a Bell inequality cannot be violated, since there exist mixed entangled states such as Werner states that can satisfy this latter condition. In theory, violation of the bound P ⩽ 0 for our steering test requires (see Methods section), while the best explicit Bell-type inequality for Werner states is violated for W ≳ 0.7056—the Vértesi bound [32] . Note this is slightly below the well-known CHSH bound of (ref. 26 ). We carefully characterized Charlie’s state preparation to determine that r *=1.081±0.009. Using a Werner state with W =0.698±0.005 (below both the CHSH and Vértesi bounds) we observed P ( r *)=0.05±0.04—a violation of our steering inequality ( Fig. 3 ). This violation may be compared with the theoretical prediction P W ( r *)=0.22 from equation (2), for ideal states and measurements. Our experimental state has a fidelity of 97.6% with a Werner state having W =0.698. Although the fidelity is high, it is not unity: our experimental state has small imperfections including an undesired population imbalance and an undesired phase shift between logical states. From modelling, we find that this accounts for the imperfection to within experimental error, with the model predicting P ( r *)=0.067. 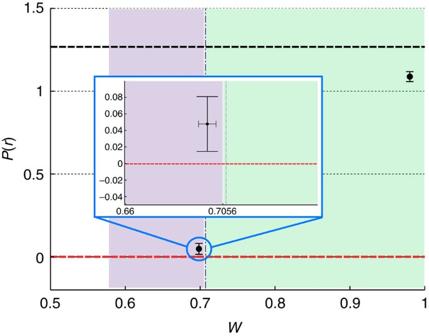Figure 3: Observed payoff function for Werner and singlet states. The main figure shows the measured values of the payoff functionP(r) forr=r*=1.081±0.009, for the cases of a Werner state withW=0.698±0.005 and a state with fidelityF≈0.98 to the ideal singlet Bell state (W=0.98). The upper dashed horizontal line indicates the maximum possible payoff,(see text), while the lower dashed horizontal line atP(r)=0 denotes the cutoff value for demonstrating steering. The purple shaded region indicates the range ofWcorresponding to steerable Werner states that do not violate any known Bell inequality, and the dot-dashed vertical line corresponds to the minimum value ofWrequired to violate the standard CHSH Bell inequality (see text). As is most clearly seen in the inset figure, the data point forW=0.698±0.005 lies to the left of the values required to violate known Bell inequalities, withP(r)>0. Hence steering is verified. The error bars are defined in the methods section. Figure 3: Observed payoff function for Werner and singlet states. The main figure shows the measured values of the payoff function P ( r ) for r = r *=1.081±0.009, for the cases of a Werner state with W =0.698±0.005 and a state with fidelity F ≈0.98 to the ideal singlet Bell state ( W =0.98). The upper dashed horizontal line indicates the maximum possible payoff, (see text), while the lower dashed horizontal line at P ( r )=0 denotes the cutoff value for demonstrating steering. The purple shaded region indicates the range of W corresponding to steerable Werner states that do not violate any known Bell inequality, and the dot-dashed vertical line corresponds to the minimum value of W required to violate the standard CHSH Bell inequality (see text). As is most clearly seen in the inset figure, the data point for W =0.698±0.005 lies to the left of the values required to violate known Bell inequalities, with P ( r )>0. Hence steering is verified. The error bars are defined in the methods section. Full size image With higher values of W (for example, W ≈1) one would also expect a verification of steering, and indeed we observed P ( r *)=1.09±0.03 for a state having a fidelity F ≈0.98 with the ideal singlet Bell state ( Fig. 3 ). This is close to the ideal value of for a singlet state, corresponding to W =1 in equation (2). Even without ideal entangled states or measuring devices, our observations of measured payoffs P ( r *)>0 meant that Charlie was able to verify that Alice could steer Bob’s state, without requiring any trust in them or their devices. EPR steering is a key quantum resource because, apart from its fundamental interest, it is known to be useful in secure quantum key distribution protocols [21] . Compared with violation of a loophole-free Bell inequality—which provides fully device-independent QKD—EPR steering in its usual form provides a one-sided device-independent protocol, requiring trust in one party (say, Bob) and their apparatus. Our demonstration of QRS removes the need to trust Bob and his apparatus, only requiring the assumption that quantum mechanics is a reliable description of reality. This lack of trust is possible essentially because Bob is unable to unambiguously distinguish between the states sent to him by Charlie [23] . Thus, as long as quantum mechanics is correct, the protocol has the advantages of Bell inequality violation, but can tolerate higher noise. It should also be noted that steering inequalities exist for an arbitrarily high degree of loss [18] , and hence corresponding QRS games can be constructed using our methods for long-distance applications such as secure quantum networks [33] . We note that the r parameter that we have introduced is only required to characterize the degree of confidence in the preparation of the referee states. It is unnecessary to characterize the state that Bob eventually receives from Charlie; indeed, transmission through any quantum channel will not change the protocol nor increase r (see Methods section). Therefore, as long as Charlie can characterize his prepared states, the protocol can proceed. Our protocol imposes a more complex measurement procedure on Bob, a joint BSM, compared with one-qubit Pauli projections required in a Bell test. As the protocol is robust against preparation and transmission imperfections of the referee states, this added complexity of Bob’s measurement is a reasonable overhead for removing all need for trust. We note that it is easier for Alice and Bob to demonstrate EPR steering to Charlie if he can prepare his states with a high degree of confidence, that is, with r ≈1. A future challenge is to demonstrate the closure of the detection loophole and space-like separation loophole for our protocol. When this is achieved, it will be possible to perform fully device-independent entanglement sharing between two parties—with only the assumption that quantum physics holds—with application in quantum key distribution, random number generation and beyond. Constructing QRS games A quantum state ρ AB on some Hilbert space H A ⊗ H B , shared between two parties Alice and Bob, is defined to be non-steerable by Alice if and only if there is a local hidden state (LHS) model for Bob [16] , that is, if and only if the joint probability of measurement outcomes a and b , for arbitrary measurements A and made by Alice and Bob, can be written in the form p ( a , b )=∑ λp ( λ ) p ( a | λ ) p ( b | λ ), with p ( b | λ ) restricted to have the quantum form . Here is the positive-operator-valued measure (POVM) corresponding to . Such LHS models, and hence non-steerable states, satisfy various EPR steering inequalities [16] , of the form where the a j denote classical random variables generated by Alice, and the B j denote quantum observables on Bob’s system. States non-steerable by Bob are similarly defined in terms of LHS models for Alice, however, we may focus on EPR steering by Alice without any loss of generality. It is known that for any EPR-steerable state shared by Alice and Bob, there is a corresponding steering inequality of the above form [34] . To construct a QRS game from any such steering inequality, we adapt a method recently used by Branciard et al . [24] for constructing games for verifying entanglement per se . In particular, for a given EPR steering inequality as in equation (3), we define a corresponding QRS game G (see Fig. 1c ) in which on each run the referee, Charlie, sends Alice a classical label j and Bob a state defined on a Hilbert space H C isomorphic to some subspace of H B . These states must be such that the equivalent states on H B form a linear basis for the observables B j , that is, for some set of coefficients g jk . Alice and Bob are not allowed to communicate during the game, but can have a prearranged strategy and perform arbitrary local operations. Alice returns a value a = a j , and Bob returns a value b =0 or 1 corresponding to some POVM on H B ⊗ H C . The corresponding payoff function is defined by P G :=∑ j , k g jk ‹ ab › j , k , where ‹·› j , k denotes the average over runs with a given j and k . Alice and Bob win the game if P G >0. The QRS game in the main text is equivalent to taking j =0, 1, 2, 3, k ≡( j , s ), a j =±1 for j =1, 2, 3, , and g jk = s (=1) for j ≠0 ( j =0). The factor of 2 in the payoff function equation (1) for this game is chosen to make P ( r ) equal to the left hand side of the steering inequality (ref. 34 ). This steering inequality can be violated for Werner states only if (ref. 34 ), and hence this condition is also necessary for Alice and Bob to be able to win the QRS game in the main text. For perfect state generation by the referee, that is, r =1 (see below), this reduces to . Note that this corresponds to the condition for a Werner state to allow EPR steering, with measurements limited to three Pauli directions, in the non-quantum-refereed scenario [16] , [17] . We now show that Alice and Bob can win game G only if Alice and Bob share a state that is EPR steerable by Alice. Restricting Alice and Bob to no communication during the game prevents them from generating a steerable state from a non-steerable one [23] , and hence we must show that if they share any non-steerable state on any Hilbert space H A ⊗ H B then P G ≤0. Now, for such a state there is some LHS model (see above), and thus where the normalization factor N , probability distribution q ( λ ) and density operator τ λ C are implicitly defined via on H C is isomorphic to B j on H B , and the average is with respect to the LHS model { τ C ( λ ); q ( λ )}. Noting the average corresponds to the left hand side of steering inequality in equation (3) for this LHS model, one has P G ≤0 as required. Conversely, analogously to the entanglement verification games of Branciard et al . [24] , it may be shown that Alice and Bob can in principle win the game if they share a state that violates the EPR steering inequality in equation (3), where Bob measures the projection B 1 onto an appropriate Bell state on H B ⊗ H C (see, for example, equation (2)). In practice, the referee cannot ensure perfect generation of the states . However, by performing tomography on these states, the referee can adjust the coefficients g jk appropriately, to take this into account. We describe one method of doing so below, for the experiment carried out in this paper, which can be easily generalized to other QRS games. We observe that it does not matter if the generated states are acted on non-trivially by some completely positive channel, φ , before reaching Bob, as this is equivalent to simply replacing Bob’s measurement on H B ⊗ H C by ( I B ⊗ φ *)( ), where φ * denotes the dual channel and I B is the identity map on H B . In particular, for the QRS game corresponding to equation (1), suppose that the referee actually generates the states . The payoff function in equation (1) then evaluates to for a shared non-steerable state, with N , q ( λ ) and defined as above and where the inequality follows using a j =±1 and v · σ ≤| v |, and we define a =( a 1 , a 2 , a 3 ), . It is straightforward to show that the right hand side of the inequality is no more than zero for r ≥ r *, with Hence, for r ≥ r *, the operator T λ ( r ) is non-positive, and hence P ( r )≤0 for any non-steerable state. It is straightforward to check that r *=1 for perfect state generation, . Determining r * experimentally involves tomographically characterizing (as below) Charlie’s state preparations { j , s } to find the Bloch vectors n ( j , s ) . We experimentally found r *=1.081±0.009. Experimental apparatus The individual spontaneous parametric downconversion (SPDC) sources used in our demonstration consisted of a pair of sandwiched bismuth borate (BiBO) crystals, each 0.5 mm in length and cut for type-I degenerate down-conversion from 410 nm (pump) to 820 nm (signal/idler), with their optic axes perpendicularly oriented. Charlie’s source was pumped with 200 mW of horizontally polarized light to generate polarization-unentangled photon pairs. One of Charlie’s photons (signal) was sent to a single-photon counting module (Perkin-Elmer SPCM-AQR-14-FC), to herald the arrival of a degenerate idler counterpart at the BSM device. The second SPDC source was pumped with 200 mW of diagonally polarized light, generating the polarization-entangled state ρ AB ≠ ρ A ⊗ ρ B shared between Alice and Bob. The state from the SPDC source could be transformed into any of the four Bell states by implementing a local unitary with a fibre polarization controller (to generate anti/correlated statistics) combined with a half-wave plate tilted in the xy plane with its optic axis in the horizontal plane (to set the phase φ of the entangled Bell state). Alice’s photon (consisting of one-half of the entangled state) was sent to her single-qubit measurement station, whereas Bob’s photon (consisting of the remaining half of the entangled state) was coupled into single-mode fibre and sent to Bob’s BSM device. Bob’s BSM device consisted of a central 50:50 beam splitter and polarization analysis at the output ports. The device combined Bob’s half of the entangled state ρ AB , and the state that Charlie sent to him. Bob’s partial BSM device resolved the |Ψ + › and |Ψ − › Bell states through discrimination of orthogonally polarized photon pairs (the case of |Ψ + ›) or through anti-bunching behaviour (the case of |Ψ − ›). On the other hand, the |Φ ± › states required number resolving detection (since these states saw pairs of photons degenerate in polarization bunched at the point of detection). Because our single-photon counting modules were not number resolving, we instead opted for pseudo-number resolution by replacing the single-mode fibres at Bob’s BSM output with single-mode 50:50 fibre beam splitters. The initially bunched pairs of photons travelling down these fibre beam splitters were separated and number-resolved 50% of the time, a feature accounted for in the analysis of the payoff function. The Bell-state analysis featured non-classical HOM interference between the ρ B and photons at the central 50:50 beam splitter. A HOM interference visibility of 89% was calculated, where a high interference visibility corresponded to effective resolution of the singlet state |Ψ − › and the other three triplet Bell states (for some local unitary). Bob performed a joint measurement on , where the fibre input coupler for the photon was kept on a linear z −translation stage to match temporal modes between the ρ B and photons. A photon detection at Alice’s detector heralded the presence of the ρ B photon at the 50:50 beam splitter, and a photon detection in Charlie’s heralding detector signified the presence of the photon. Our method to calculate the payoff function P ( r ) for an experimental Werner state ρ AB was relatively straightforward, and used the fact that a Werner state can be expressed as a statistical mixture of all four Bell states. Data was taken with ρ AB consecutively prepared in the four Bell states, and the data sets were aggregated to produce a value of the payoff function for the effective state ρ AB . The Werner parameter was tuned by weighting the data collection time for the singlet state relative to the data collection time for the three triplet states (where the data collection interval for the three triplet states was identical). For example, to test the payoff function using a completely mixed state ( W =0), data could be taken for an equal time with all four Bell states. Taking a relatively shorter collection time for the triplet states allowed us to obtain a mixture corresponding to a Werner state with W =0.0698±0.005, below the CHSH and Vértesi bounds for Bell inequality violation by a Werner state (see main text). It may be remarked that it remains an open question whether there exists a Bell inequality that can be violated for W below the Vértesi bound, although it is known to be impossible for W ≲ 0.6595 (refs 32 , 35 ). Charlie’s ability to send the correct state to Bob was also experimentally characterized. An average fidelity of av =98.7±0.6% was measured in the Bell-state analysis set-up for the six Pauli operator eigenstates prepared by Charlie’s source. All states were characterized using maximum-likelihood quantum state tomography as per ref. 36 , and fidelities between (in general) mixed states ρ and σ given by the standard formula . Experimental error analysis Experimental uncertainties were derived from Poissionian counting statistics and standard error propagation techniques. Error bars quoted represent ±1 standard deviations. Where uncertainties are required in quantities derived from tomographic state reconstructions [36] , the process was as follows. A large number of tomographic reconstructions on the state were performed, with each trial drawing from a Poissonian distribution of statistics for each measurement outcome. Each of the reconstructed density matrices were used to calculate the parameter of interest (for example, W ), and the mean and s.d. of the distribution in that parameter produced the value and its uncertainty. How to cite this article : Kocsis, S. et al . Experimental measurement-device-independent verification of quantum steering. Nat. Commun. 6:5886 doi: 10.1038/ncomms6886 (2015).